Food restriction enhances visual cortex plasticity in adulthood Neural circuits display a heightened sensitivity to external stimuli during well-established windows in early postnatal life. After the end of these critical periods, brain plasticity dramatically wanes. The visual system is one of the paradigmatic models for studying experience-dependent plasticity. Here we show that food restriction can be used as a strategy to restore plasticity in the adult visual cortex of rats. A short period of food restriction in adulthood is able both to reinstate ocular dominance plasticity and promote recovery from amblyopia. These effects are accompanied by a reduction of intracortical inhibition without modulation of brain-derived neurotrophic factor expression or extracellular matrix structure. Our results suggest that food restriction could be investigated as a potential way of modulating plasticity. Nutrition is a fundamental component of our life. The quality and quantity of food consumed by each individual is critical for the development and maintenance of its general physical structure. A great number of studies have identified several specific dietary components that are essential for the correct development of the central nervous system [1] . Interestingly, it has been demonstrated that simply reducing the caloric intake can lead to an extension of the mean and maximum life span in a wide range of organisms, including yeasts, worms, fruit flies, rodents and monkeys [2] . This increase in longevity is often accompanied by an effective counteraction of the aging process both at the level of body healthness with reduced incidence of age-related cardiomyopathy, diabetes, hypertension and neoplastic processes [3] , [4] , and at the level of brain physiology. Noteworthy, various protocols of food restriction (FR) delay the onset of learning and memory decline leading to an improvement of animal performances in behavioural tests [5] , [6] and suppressing synaptic deficits in the hippocampus [7] , [8] . These effects could involve neural plasticity processes. We directly addressed this issue exploiting the visual cortex as a testing system. The ocular dominance (OD) shift of cortical neurons in response to the closure of one eye (monocular deprivation, MD) is the most classic experimental paradigm for studying experience-dependent plasticity. Long-term MD in animal models induces amblyopia, a pathological condition characterized by a loss of visual acuity (VA) in the affected eye and a pronounced OD shift of visual cortical neurons in favour of the normal eye. Visual circuits are highly sensitive to environmental stimuli only during developmental time windows with a dramatic decline of plasticity in adulthood [9] . Similarly, it is currently accepted that the recovery from amblyopia is possible only early in the development. In this study, we tested whether FR could restore plasticity in the adult visual cortex. We found that reduction in caloric intake triggered both a full OD shift following MD and a complete recovery from amblyopia in adult animals. We also report that a reduction of intracortical inhibition and an increase in histone acetylation accompanied this plastic outcome. Physiological response to food restriction in adult rats Adult rats (>P60) were subjected to a widely used protocol of FR consisting of a fasting regimen on alternate days with maintenance of the composition of the diet in terms of vitamins, minerals and proteins. In other words, the animals had no access to food for a full day, every other day, whereas they were allowed to eat ad libitum on the intervening days. After 4 weeks of this dietary regimen (P60–P90), food-restricted rats (FR rats) showed a reduction of about 22% in the daily food assumption ( Fig. 1a ). The body weight of FR rats was lower than controls (CTLs), the reduction being present since the first week of diet. At the end of the fourth week of FR, mean body weight of restricted rats decreased by about 10% with respect to CTLs ( Fig. 1b ). 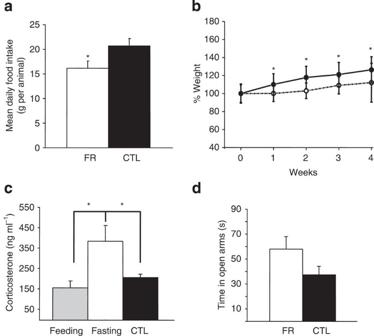Figure 1: Effects of food restriction on body physiology and stress behaviour in food-restricted rats. (a) Food intake was measured in the last 10 days of diet. Food intake of food-restricted rats (FR;n=6; mean daily food intake 16.15±1.47 g) was significantly lower with respect to controls (CTL,n=6; mean daily food intake 20.67±1.52 g; two-way ANOVAP<0.001). (b) Body weight measured during the whole period of dietetic regimen showed a significant reduction in the FR animals (solid line) with respect to CTLs (dashed line) since the first week of diet. At the end of treatment, mean body weight of FR rats was 112.06±21.56% of the initial value, whereas mean body weight of CTLs was 126.31±14.55% of their initial value. The difference between the two groups was always statistically significant (FRn=6; CTLn=6; two-way ANOVAP<0,001). (c) Serum content of corticosterone in FR animals and CTLs. Samples from each animal were collected at the same time of the day, that is, at the beginning of the active phase (1700 hours). In FR rats (n=6), corticosterone levels were significantly higher with respect to CTLs (n=10) at the end of a fasting day (383.75±77.5 versus 205.09±17.05 ng ml−1;t-testP=0.026), whereas they returned to normality after 1 day of feeding (n=7; 155.10±34.25 ng ml−1; feeding versus CTLst-testP=0.173). (d) In the elevated plus maze test, FR rats (n=6) spent the same time in open arms with respect to CTLs (n=6; 58±10 versus 37±7 s;t-testP=0.123). Error bars represent s.e.m.; asterisks indicate statistical significance. Figure 1: Effects of food restriction on body physiology and stress behaviour in food-restricted rats. ( a ) Food intake was measured in the last 10 days of diet. Food intake of food-restricted rats (FR; n =6; mean daily food intake 16.15±1.47 g) was significantly lower with respect to controls (CTL, n =6; mean daily food intake 20.67±1.52 g; two-way ANOVA P <0.001). ( b ) Body weight measured during the whole period of dietetic regimen showed a significant reduction in the FR animals (solid line) with respect to CTLs (dashed line) since the first week of diet. At the end of treatment, mean body weight of FR rats was 112.06±21.56% of the initial value, whereas mean body weight of CTLs was 126.31±14.55% of their initial value. The difference between the two groups was always statistically significant (FR n =6; CTL n =6; two-way ANOVA P <0,001). ( c ) Serum content of corticosterone in FR animals and CTLs. Samples from each animal were collected at the same time of the day, that is, at the beginning of the active phase (1700 hours). In FR rats ( n =6), corticosterone levels were significantly higher with respect to CTLs ( n =10) at the end of a fasting day (383.75±77.5 versus 205.09±17.05 ng ml −1 ; t -test P =0.026), whereas they returned to normality after 1 day of feeding ( n =7; 155.10±34.25 ng ml −1 ; feeding versus CTLs t -test P =0.173). ( d ) In the elevated plus maze test, FR rats ( n =6) spent the same time in open arms with respect to CTLs ( n =6; 58±10 versus 37±7 s; t -test P =0.123). Error bars represent s.e.m. ; asterisks indicate statistical significance. Full size image Most studies on FR have shown that a reduction in the caloric intake is accompanied by an increase in the serum levels of corticosterone [10] , [11] , [12] , [13] , a body homeostatic response to the need for enhanced glicogenolysis. In FR rats, we observed almost a 100% increase in the blood content of corticosterone. Noteworthy, this increase was present only at the end of a fasting day, whereas corticosterone levels returned to normality after 1 day of feeding ( Fig. 1c ). The elevation of plasma corticosterone indicates that FR could cause a period of stress in the animals. Nevertheless, it has been suggested that FR represents only a low-intensity stressor, as the FR-induced elevation of plasma-free corticosterone is generally smaller compared with other stressing experimental protocols, such as restraint, which causes a rapid, marked elevation of plasma corticosterone and a disregulation of the hypothalamic–pituitary–adrenal axis [14] . Accordingly, we found that FR rats did not show any increase in mean daily locomotor activity with respect to CTLs and, when subjected to the elevated plus maze test (a validated method to measure anxiety-like behaviours in rodents [15] ), they displayed a performance very similar to the CTL group ( Fig. 1d ). Restoration of visual cortex plasticity in adult rats To assess whether reducing the caloric intake could restore visual cortex plasticity in adulthood, we used two classical models of visual system plasticity: the OD shift of cortical neurons after MD and the recovery from amblyopia after reverse suture (RS). The effectiveness of these two manipulations in the rat is restricted to the CP. To test whether 7 days of MD were effective in shifting the OD distribution (binocularity) of adult FR rats, the animals were monocularly deprived during the last week of the dietetic regimen. We evaluated OD distribution in the binocular portion of the primary visual cortex (V1) contralateral to the occluded eye by measuring the contra-ipsi (C/I) visual evoked potential (VEP) ratio, that is, the ratio between the responses elicited by the stimulation of the two eyes (see Methods). The C/I VEP ratio is in the range of 2–3 in adult normal animals, whereas it is strongly reduced ( ∼ 1) in rats subjected to MD during the CP. As expected, 1 week of MD did not affect the C/I VEP ratio in the visual cortex of CTL adult animals, confirming the absence of OD plasticity in adult rats (C/I VEP ratio=2.81±0.21; n =5; Fig. 2a ). When MD was performed in FR rats, however, we observed a marked OD shift in favour of the non-deprived eye, reflected by a significant decrease of the C/I VEP ratio (C/I VEP ratio=1.29±0.21; n =8; t -test, P <0.001; Fig. 2a ). We also measured VA of both eyes by using VEP recordings in the visual cortex contralateral to the closed eye and, also in this case, we found that the responsiveness to MD was reinstated in FR rats. The VA of the deprived eye, indeed, was significantly reduced with respect to the open eye in FR rats (0.86±0.05 versus 1.04±0.04 c deg −1 ; n =6; paired t -test P =0.027; Fig. 2b ), whereas the VA of the two eyes was comparable in CTL animals (0.92±0.03 versus 0.95±0.04 c deg −1 ; n =6; paired t -test P =0.385). 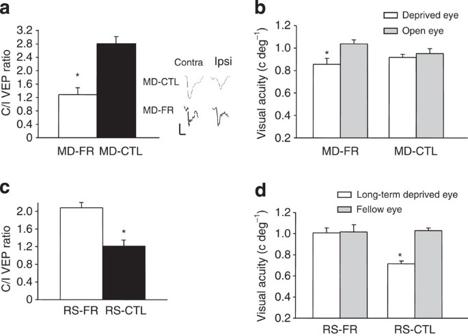Figure 2: Restoration of visual cortex plasticity in animals. (a) OD was measured after 7 days of monocular deprivation in food-restricted rats (MD-FR, C/I VEP ratio=1.29±0.21;n=8) and in controls (MD-CTL, C/I VEP ratio=2.81±0.21;n=5;t-test,P<0.001). (b) Similarly, VA of the deprived eye and of the fellow non-deprived eye was evaluated both in MD-FR rats (0.86±0.05 versus 1.04±0.04 c deg−1;n=6; pairedt-testP=0.027) and in MD-CTL animals (0.92±0.03 versus 0.95±0.04 c deg−1;n=6; pairedt-testP=0.385) after 7 days of MD. (c) Analysis of binocularity was carried out in the visual cortex contralateral to the long-term deprived eye through VEP ratio measurement in food-restricted, reverse-sutured rats (RS-FR, C/I VEP ratio=2.08±0.12;n=7) and in controls (RS-CTL, C/I VEP ratio=1.21±0.14;n=6;t-test,P<0.001). (d) Recovery of VA in the formerly deprived eye was evaluated in RS-FR rats (1.01±0.05 versus 1.02±0.07 c deg−1;n=5; pairedt-testP=0.851) and in RS-CTL animals (0.72±0.03 versus 1.03±0.02 c deg−1;n=4; pairedt-testP=0.004). Error bars represent s.e.m.; asterisks indicate statistical significance. Figure 2: Restoration of visual cortex plasticity in animals. ( a ) OD was measured after 7 days of monocular deprivation in food-restricted rats (MD-FR, C/I VEP ratio=1.29±0.21; n =8) and in controls (MD-CTL, C/I VEP ratio=2.81±0.21; n =5; t -test, P <0.001). ( b ) Similarly, VA of the deprived eye and of the fellow non-deprived eye was evaluated both in MD-FR rats (0.86±0.05 versus 1.04±0.04 c deg −1 ; n =6; paired t -test P =0.027) and in MD-CTL animals (0.92±0.03 versus 0.95±0.04 c deg −1 ; n =6; paired t -test P =0.385) after 7 days of MD. ( c ) Analysis of binocularity was carried out in the visual cortex contralateral to the long-term deprived eye through VEP ratio measurement in food-restricted, reverse-sutured rats (RS-FR, C/I VEP ratio=2.08±0.12; n =7) and in controls (RS-CTL, C/I VEP ratio=1.21±0.14; n =6; t -test, P <0.001). ( d ) Recovery of VA in the formerly deprived eye was evaluated in RS-FR rats (1.01±0.05 versus 1.02±0.07 c deg −1 ; n =5; paired t -test P =0.851) and in RS-CTL animals (0.72±0.03 versus 1.03±0.02 c deg −1 ; n =4; paired t -test P =0.004). Error bars represent s.e.m. ; asterisks indicate statistical significance. Full size image We next evaluated whether this potential for plasticity could be exploited for restoring normal visual functions in adult amblyopic animals. Rats rendered amblyopic by long-term MD starting from P21 were subjected to FR protocol in adulthood (1 month starting at P60) and RS was performed during the last 2 weeks of diet. In adult FR rats, binocularity (C/I VEP ratio=2.08±0.12; n =7) and VA of the amblyopic eye (VA of long-term deprived eye=1.01±0.05 c deg −1 , VA of not occluded eye=1.02±0.07 c deg −1 ; n =5; paired t -test P =0.851) exhibited a complete rescue. In contrast, we did not observe any sign of recovery in CTL animals (C/I VEP ratio=1.21±0.14; n =6; VA of long-term deprived eye=0.72±0.03 c deg −1 ; VA of not occluded eye=1.03±0.02 c deg −1 ; n =4; paired t -test P =0.004; Fig. 2c,d ). FR regulates inhibition levels in the adult visual cortex Inhibition is well known to have a crucial role in the expression and regulation of neural plasticity during development and adulthood: there is evidence, indeed, that the inhibitory tone is essential for the time course of critical period in the visual cortex [16] and it has been demonstrated that strategies decreasing inhibition reactivate developmental levels of plasticity in the adult brain [17] . We quantified the extracellular levels of γ-aminobutyric acid (GABA) and glutamate in the binocular visual cortex of FR and CTL animals using in vivo brain microdialysis and high-performance liquid chromatography (HPLC). Extracellular GABA levels were significantly reduced in the visual cortex FR rats with respect to CTLs (0.51±0.12 versus 2.94±0.33 pmol μl −1 ; FR n =7; CTLs n =6; t -test P <0.001; Fig. 3a ), whereas no differences in glutamate levels were detected ( Supplementary Fig. S1 ). 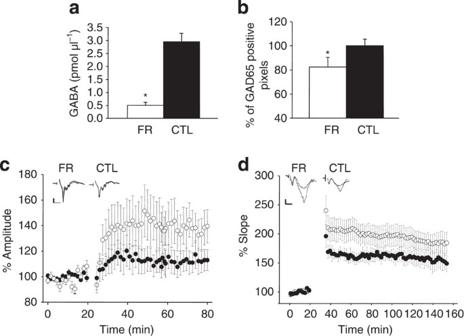Figure 3: Reduction of intracortical inhibition in the visual cortex and increased synaptic plasticity following food restriction. (a) Measurement of GABA release in the visual cortex of food-restricted rats (FR=0.51±0.12 pmol μl−1;n=7;t-testP<0.001) with respect to controls (CTL=2.94±0.33 pmol μl−1;n=5) usingin vivobrain microdialysis. (b) GAD65 expression was quantified through immunohistochemistry in the visual cortex of FR rats (n=6) and in CTLs (n=6;t-testP=0.001). (c) Average time course of layer II–III field potential (FP) amplitude before and after θ-burst stimulation of white matter (WM). White circles represent averaged field potential from FR rats (n=7 slices, 5 animals; two-way RM ANOVA, baseline versus the last 20 min of post-theta,P=0.025), whereas filled circles represent data from CTLs (n=7 slices, 5 animals; two-way RM ANOVA, baseline versus the last 20 min of post-theta,P=0.218). The difference between post-theta response in FR animals and CTLs was also evaluated (two-way ANOVA in the last 20 min of post-theta,P<0.001). A dot is the result of the average of three different measurements, each taken every 30 s. Waveform examples are represented. Vertical calibration bar, 100 μV; horizontal calibration bar, 2 ms. (d) LTP in the CA1 subfield of the hippocampus was induced through stimulation of Schaffer collaterals and time course of FP slope was recorded before and after high-frequency stimulation. Results from FR rats (white circles;n=6 slices, 5 animals; two-way RM ANOVA, baseline versus the last 20 min of post-theta,P=0.004) and CTLs (filled circles;n=4 slices, 3 animals; two-way RM ANOVA, baseline versus the last 20 min of post-theta,P=0.049) are illustrated. The difference between LTP in FR animals and CTLs was also measured (two-way ANOVA in the last 20 min of post-theta,P<0.001). A dot is the result of the average of four different measurements, each taken every 30 s. Examples of waveforms from hippocampal slices are represented. Vertical calibration bar, 500 μV; horizontal calibration bar, 2 ms. Error bars represent s.e.m.; asterisks indicate statistical significance. Figure 3: Reduction of intracortical inhibition in the visual cortex and increased synaptic plasticity following food restriction. ( a ) Measurement of GABA release in the visual cortex of food-restricted rats (FR=0.51±0.12 pmol μl −1 ; n =7; t -test P <0.001) with respect to controls (CTL=2.94±0.33 pmol μl −1 ; n =5) using in vivo brain microdialysis. ( b ) GAD65 expression was quantified through immunohistochemistry in the visual cortex of FR rats ( n =6) and in CTLs ( n =6; t -test P =0.001). ( c ) Average time course of layer II–III field potential (FP) amplitude before and after θ-burst stimulation of white matter (WM). White circles represent averaged field potential from FR rats ( n =7 slices, 5 animals; two-way RM ANOVA, baseline versus the last 20 min of post-theta, P =0.025), whereas filled circles represent data from CTLs ( n =7 slices, 5 animals; two-way RM ANOVA, baseline versus the last 20 min of post-theta, P =0.218). The difference between post-theta response in FR animals and CTLs was also evaluated (two-way ANOVA in the last 20 min of post-theta, P <0.001). A dot is the result of the average of three different measurements, each taken every 30 s. Waveform examples are represented. Vertical calibration bar, 100 μV; horizontal calibration bar, 2 ms. ( d ) LTP in the CA1 subfield of the hippocampus was induced through stimulation of Schaffer collaterals and time course of FP slope was recorded before and after high-frequency stimulation. Results from FR rats (white circles; n =6 slices, 5 animals; two-way RM ANOVA, baseline versus the last 20 min of post-theta, P =0.004) and CTLs (filled circles; n =4 slices, 3 animals; two-way RM ANOVA, baseline versus the last 20 min of post-theta, P =0.049) are illustrated. The difference between LTP in FR animals and CTLs was also measured (two-way ANOVA in the last 20 min of post-theta, P <0.001). A dot is the result of the average of four different measurements, each taken every 30 s. Examples of waveforms from hippocampal slices are represented. Vertical calibration bar, 500 μV; horizontal calibration bar, 2 ms. Error bars represent s.e.m. ; asterisks indicate statistical significance. Full size image To further analyse the effects of FR on the GABAergic system, the expression of GAD65 in the visual cortex of FR and controls animals was assessed by means of semi-quantitative immunohistochemistry. GAD65 is the 65-kDa isoform of the enzyme responsible for GABA synthesis (glutamic acid decarboxylase), whose expression is more prominent at synaptic level [18] . We found that puncta-ring immunoreactivity (see Methods) of GAD65 was significantly reduced in FR rats as compared with CTLs ( t -test P =0.001; Fig. 3b ). Potentiation of cortical and hippocampal synaptic plasticity Maturation of inhibition has been proposed to reduce synaptic plasticity in the visual cortex by acting as a gate, which filters the level and pattern of activity that layer IV, the major thalamo-recipient layer, is able to relay to supragranular layers [19] , [20] , [21] . Indeed, it has been demonstrated that the induction of long-term potentiation (LTP) in the layer II–III of the cortex through stimulation of the white matter (WM-LTP) declines with age and contrasting inhibition by acute application of GABA receptor antagonists on visual cortical slices in adulthood enhances WM-LTP [22] . Given these results, we tested whether the reduction of inhibition observed in adult FR rats was sufficient to restore WM-LTP in the visual cortex. As expected, LTP induction was absent in CTL animals, whereas visual cortical slices taken from FR rats showed a robust potentiation of field potential (FP) amplitudes after WM stimulation (FR n =7 slices, 5 animals; CTLs n =7 slices, 5 animals; two-way analysis of variance (ANOVA) FR versus CTLs P <0.001; Fig. 3c ). Noteworthy, FR also increased LTP expression induced by Schaffer collateral stimulation in the CA1 hippocampal subfield (FR n =6 slices, 5 animals; CTLs n =4 slices, 3 animals; two-way ANOVA FR versus CTLs P <0.001; Fig. 3d ), demonstrating that the facilitation of synaptic plasticity was not confined to the visual cortex. No difference in the excitability of FR slices with respect to CTLs was found in either visual cortex or hippocampus ( Supplementary Fig. S2 ). Benzodiazepine treatment prevents restoration of plasticity It has been recently demonstrated that pharmacological treatment with mercaptopropionic acid or picrotoxin is effective in reducing inhibition and restoring plasticity to the visual cortex of adult rats [23] . These results were comparable to those obtained with FR ( Supplementary Fig. S3 ). To analyse how crucial was the role of decreased inhibition for the effects obtained in FR rats, we artificially strengthened GABAergic transmission in a separate group of FR animals by cortical infusion via osmotic minipumps of the benzodiazepine agonist diazepam. Diazepam enhances GABA receptor-mediated current, and is a common tool used for enhancing inhibition in the cerebral cortex [16] . We measured binocularity in monocularly deprived FR rats treated with diazepam by recording C/I VEP ratio in the visual cortex contralateral to the deprived eye. Diazepam infusion prevented the decrease of C/I VEP ratio due to FR (2.03±0.14; n =6; t -test on rank P =0.02; Fig. 4a ). Moreover, VA of the deprived eye was normal in FR animals intracortically infused with diazepam and did not differ from VA of the open eye (VA of the deprived eye=0.95±0.05 c deg −1 ; VA of the open eye 1.00±0.02 c deg −1 ; t -test P =0.505; Fig. 4b ). These results demonstrate that the decrease of intracortical inhibition has a pivotal role for the restoration of visual cortex plasticity induced by FR. 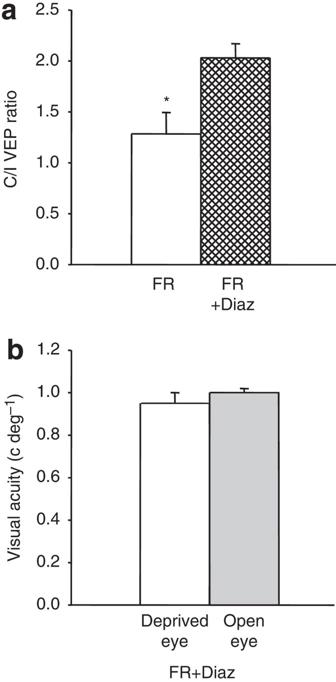Figure 4: Restoration of plasticity is prevented by benzodiazepines treatment. (a) The C/I VEP ratio of control (CTL) animals was compared with the VEP ratio of FR rats treated with diazepam and monocularly deprived for one week (FR+Diaz, 2.03±0.14;n=6;t-testP=0.02). (b) Visual acuity of the deprived eye and of the open eye in FR+Diaz rats (0.95±0.05 versus 1.00±0.02 c deg−1; pairedt-testP=0.505). Error bars represent s.e.m.; asterisk indicates statistical significance. Figure 4: Restoration of plasticity is prevented by benzodiazepines treatment. ( a ) The C/I VEP ratio of control (CTL) animals was compared with the VEP ratio of FR rats treated with diazepam and monocularly deprived for one week (FR+Diaz, 2.03±0.14; n =6; t -test P =0.02). ( b ) Visual acuity of the deprived eye and of the open eye in FR+Diaz rats (0.95±0.05 versus 1.00±0.02 c deg −1 ; paired t -test P =0.505). Error bars represent s.e.m. ; asterisk indicates statistical significance. Full size image Corticosterone mimics FR effects on visual cortex plasticity It has been hypothesized that exposure to mild stressors activates homeodynamic pathways of maintenance and repair triggering beneficial effects on brain functions [24] . Indeed, although high levels or chronic stress have been associated with reduced synaptic plasticity in the hippocampus, a mild or acute stress has been demonstrated to increase LTP induction [25] . Given its well-known involvement in stress response, corticosterone could emerge as a candidate for regulating processes of experience-dependent plasticity triggered by FR. We addressed this issue pharmacologically mimicking the every other day elevation of blood corticosterone caused by our protocol of FR. We treated a group of rats with a low dose of corticosterone in drinking water on alternate days for 4 weeks, as previously reported in rodents [26] , [27] , [28] , and we tested visual cortex plasticity evaluating the effects of 1 week of MD on OD distribution of cortical neurons. We found a significant shift of C/I VEP ratio in favour of the open eye in the visual cortex of MD rats treated with corticosterone (C/I VEP ratio=1.22±0.07; n =5; one-way ANOVA P <0.001; post hoc Holm–Sidak test CTL versus FR P <0.001; CTL versus Cort P <0.001; Cort versus FR P =0.826; Fig. 5a ), as well as a decrease of the deprived-eye VA (VA of the deprived eye=0.75±0.02 c deg −1 ; VA of the open eye=1.00±0.02; paired t -test P <0.001; Fig. 5b ). 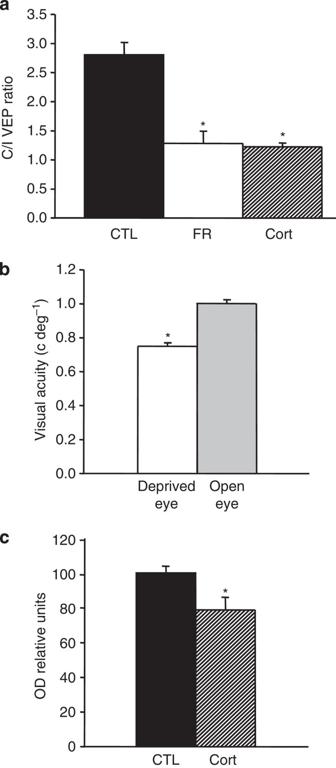Figure 5: Corticosterone treatment restores plasticity in adult rats. (a) Assessment of C/I VEP ratio in control (CTL) and in adult MD rats treated with corticosterone on alternate days (Cort, C/I VEP ratio=1.22±0.07;n=5; one-way ANOVAP<0.001;post hocHolm–Sidak test CTL versus FRP<0.001; CTL versus CortP<0.001; Cort versus FRP=0.826). (b) Visual acuity of the two eyes in MD animals treated with corticosterone (VA of the deprived eye=0.75±0.02 c deg−1; VA of the open eye=1.00±0.02; pairedt-testP<0.001). (c) Western blot analysis was used to evaluate GAD65 expression in adult animals treated with corticosterone on alternate days with respect to controls (n=5 Cort;n=11 CTL;t-testP=0.015). Error bars represent s.e.m.; asterisks indicate statistical significance. Figure 5: Corticosterone treatment restores plasticity in adult rats. ( a ) Assessment of C/I VEP ratio in control (CTL) and in adult MD rats treated with corticosterone on alternate days (Cort, C/I VEP ratio=1.22±0.07; n =5; one-way ANOVA P <0.001; post hoc Holm–Sidak test CTL versus FR P <0.001; CTL versus Cort P <0.001; Cort versus FR P =0.826). ( b ) Visual acuity of the two eyes in MD animals treated with corticosterone (VA of the deprived eye=0.75±0.02 c deg −1 ; VA of the open eye=1.00±0.02; paired t -test P <0.001). ( c ) Western blot analysis was used to evaluate GAD65 expression in adult animals treated with corticosterone on alternate days with respect to controls ( n =5 Cort; n =11 CTL; t -test P =0.015). Error bars represent s.e.m. ; asterisks indicate statistical significance. Full size image Interestingly, western blot analysis revealed a reduction of GAD65 levels in the visual cortex of rats treated with corticosterone ( n =11 CTL; n =5 Cort; t -test P =0.015; Fig. 5c ), suggesting that the enhancement of corticosterone levels due to FR could be involved in the modulation of intracortical excitation–inhibition balance. Extracellular matrix remodelling and neurotrophin expression Restoration of plasticity in the adult has been often associated with increased levels of neurotrophins and remodelling of extracellular matrix [29] , [30] , [31] , [32] . We tested whether FR affected brain-derived neurotrophic factor (BDNF) content in the adult visual cortex by means of immunohistochemistry and western blot. No difference in BDNF was detectable between the two groups using both methods ( Fig. 6a,b ). Similarly, immunohistochemistry for Wisteria Floribunda (WFA, an effective marker of CSPGs which are major components of PNNs) did not show any difference between FR rats and CTLs ( Fig. 6c ). Thus, we conclude that a short-term protocol of FR is unable to induce changes in BDNF expression or perineuronal nets composition. 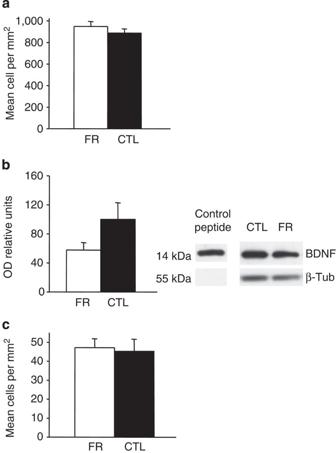Figure 6: Levels of BDNF protein and WFA in the visual cortex of adult food-restricted rats and controls. (a) Immunohistochemistry for BDNF in food-restricted rats (FR; cell density 949±46 cell per mm2;n=6) and control (CTL; cell density 888±38 cell per mm2;n=6;t-testP=0.330). (b) Analysis of BDNF protein by means of western blot in FR animals (n=4) and control rats (n=4;t-testP=0.145). (c) Density of WFA-labelled cells was measured in the two experimental groups by means of immunohistochemistry (cell density in FR rats 47±5 cell per mm2,n=6; cell density in controls 45±6 cell per mm2,n=6;t-testP=0.812). Error bars represent s.e.m. β-tub, β-tubulin. Figure 6: Levels of BDNF protein and WFA in the visual cortex of adult food-restricted rats and controls. ( a ) Immunohistochemistry for BDNF in food-restricted rats (FR; cell density 949±46 cell per mm 2 ; n =6) and control (CTL; cell density 888±38 cell per mm 2 ; n =6; t -test P =0.330). ( b ) Analysis of BDNF protein by means of western blot in FR animals ( n =4) and control rats ( n =4; t -test P =0.145). ( c ) Density of WFA-labelled cells was measured in the two experimental groups by means of immunohistochemistry (cell density in FR rats 47±5 cell per mm 2 , n =6; cell density in controls 45±6 cell per mm 2 , n =6; t -test P =0.812). Error bars represent s.e.m. β-tub, β-tubulin. Full size image FR promotes histone acetylation in V1 and hippocampus Finally, we analysed the level of histone H3 acetylation in the visual cortex and hippocampus of adult animals subjected to FR using Lys 9 acetyl-H3 (AcH3)-specific antibodies in western blot experiments. Histone post-translational modifications regulate chromatin susceptibility to transcription with high levels of histone acetylation on a specific DNA segment being generally correlated with increased transcription rates [33] , [34] . Visual experience activates histone acetylation in the visual cortex during the critical period, but this capacity is downregulated in adult animals [35] , [36] , [37] . We found that FR regimen induced a pronounced increase in H3 acetylation in the visual cortex (FR n =6; CTLs n =6; t -test P =0.048). A similar effect was evident also in the hippocampus (FR n =8; CTLs n =8; t -test P =0.046; Fig. 7 ). More specifically, we reported that the enhancement of histone acetylation in FR rats was in the range of 50–60% in the visual cortex, whereas it was of about 100% in the hippocampus. 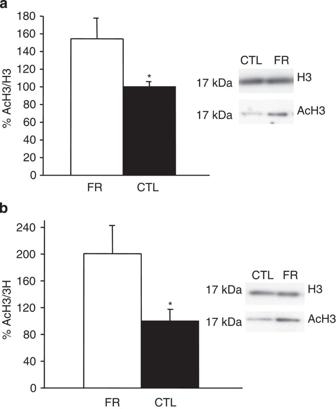Figure 7: Food restriction induced sustained H3 Lys 9 acetylation. The ratio between the intensity of the bands of AcH3 and total H3 was used as an index of the amount of acetylated H3. (a) Analysis of histone acetylation in the visual cortex of food-restricted (FR) rats with respect to controls (FR animalsn=6; CTL animalsn=6;t-testP=0.048). (b) Comparison of histone acetylation in the hippocampus of FR and control animals (FR animalsn=8; CTL animalsn=8;t-testP=0.046). Error bars represent s.e.m.; asterisks indicate statistical significance. Figure 7: Food restriction induced sustained H3 Lys 9 acetylation. The ratio between the intensity of the bands of AcH3 and total H3 was used as an index of the amount of acetylated H3. ( a ) Analysis of histone acetylation in the visual cortex of food-restricted (FR) rats with respect to controls (FR animals n =6; CTL animals n =6; t -test P =0.048). ( b ) Comparison of histone acetylation in the hippocampus of FR and control animals (FR animals n =8; CTL animals n =8; t -test P =0.046). Error bars represent s.e.m. ; asterisks indicate statistical significance. Full size image The capability to survive food deprivation is considered to be a primitive advantageous adaptation [38] , a component of the homeodynamic response of living systems to environmental changes [14] . We show that a short-term protocol of FR starting in adulthood is able to restore neural plasticity in the visual system with a rescue of the juvenile-like responsiveness to MD and a renewed capability in inducing WM-LTP in the visual cortex. The latter result is not limited to the visual system, the enhancement of synaptic plasticity being also present in the hippocampus. We suggest that the dietary regimen has a general impact on brain function and that reducing the caloric intake promotes experience-dependent modifications of neuronal circuits in adulthood. Interestingly, the increase in plasticity is also effective in the treatment of amblyopia, as FR amblyopic rats show a complete recovery of visual functions (binocularity and VA) after RS. The cellular and molecular mechanisms underlying the effects of dietary restriction are so far unclear. In the last few years, the excitation–inhibition balance in the brain has been increasingly recognized as a crucial hub for the restoration of plasticity in the adult nervous system [39] . It has been demonstrated that the pharmacological or physiological reduction of inhibition in the visual cortex of adult rats is sufficient to restore OD shift in response to MD [23] , [30] , [31] , [32] . Here, we show that FR is associated with a marked reduction of GABAergic inhibition, as evaluated using both biochemical and electrophysiological methods, and we also provide evidence that an artificial increase of inhibition in the visual cortex by infusion of the benzodiazepine diazepam prevents the OD shift due to MD in FR rats. These findings further confirm that the reduction of intracortical inhibitory transmission has a fundamental role for reopening plasticity in the adult nervous system. Restriction of caloric intake has been associated with an increase in the peak concentration of plasma corticosterone [10] , [11] , [12] , [13] . Moreover, it has been suggested that stress-induced elevations in glucocorticoid levels modulate hippocampal plasticity according to an inverted U-shaped function, with a moderate amount of circulating glucocorticoid-facilitating LTP expression, whereas higher glucocorticoid concentration impairing synaptic plasticity [40] . We observed an enhancement in the corticosterone blood content of FR animals only at the end of the fasting day. In addition, we show that an artificial increase of corticosterone levels on alternating days, mimicking that obtained with FR, does, indeed, reinstate OD plasticity in the visual cortex. Noteworthy, this treatment produced a similar reduction of GAD65 expression in the visual cortex with respect to FR. In agreement with our results, it has been recently suggested that acute stress can reduce GABA release and inhibitory post-synaptic potential (IPSP) currents in the hippocampus [41] , [42] . We demonstrate that FR is also associated with an elevation in the rate of histone acetylation both in the visual cortex and in the hippocampus. Consistently, it has been previously demonstrated that the use of histone deacetylase inhibitors causes a life span extension [43] and an increase in adult brain plasticity [35] , [36] , [37] . Our results are quite similar to those obtained with other protocols, including environmental enrichment, both at the level of functional reactivation of plasticity in adulthood [30] , [32] and at the level of increase in histone acetylation [44] . In spite of this, some of the molecular mechanisms associated with recovery of plasticity in environmental enrichment and FR seem to be different. FR animals, indeed, did not show any change in BDNF expression. This result is particularly unexpected and could be due to the short protocol of dietetic regimen adopted. In accordance with this hypothesis, it has been reported that a brief period of FR after spinal chord injury is not associated with cortical or spinal chord enhancement of BDNF [45] . In all works showing an increase in BDNF signalling after FR, either adult animals restricted for 3 months or aged mice maintained under dietary regimen for their whole life were used [46] , [47] , [48] , [49] . Our results suggest that FR could restore plasticity in the adult visual system along pathways, which are different, at least in part, from those observed with other protocols. These pathways, however, may converge on chromatin remodelling, which could be the final step in the process of plasticity induction. Animal housing and dietary regimen A total of 113 Long-Evans hooded rats of both genders, aged between P60 and P90, were used in this study, approved by the Italian Ministry of Public Health. Animals were reared in a standard cages (40×30×20 cm 3 ), housing a maximum of three adult rats. Animals were maintained at a temperature of 20–22 °C under a 12-h light/dark cycle and had ad libitum access to water. At P60, animals were randomly divided into two 'nutritional' groups: an ad libitum group (CTL) with unlimited access to food, and a FR group consisting of animals with access to food only on alternate days. The total duration of the dietary regimen was 4 weeks for all the animals. Once a week the animals were weighted, and in the last 10 days of dietetic regimen food intake was measured. All the animals had access to a standard diet (see Supplementary Methods for details). Animal treatment and drug administration After 3 weeks of treatment, rats were anaesthetized with avertin (2,2,2 tribromoethanol in amylene hydrate; 1 ml per hg of body weight, i.p). MD was performed through eyelid suturing and the animals were returned to their respective housing conditions. In different groups of rats, during the same anaesthesia, an osmotic minipump (model 2002; Alzet) connected via polyethylene (PE) tubing to a stainless steel cannula (30 gauge) was implanted in the visual cortex contralateral to the deprived eye. Osmotic minipumps (flow rate, 0.5 μl h −1 ) were filled with diazepam (2 mg ml −1 in 50% propylene glycol) or mercaptopropionic acid (100 μM; Sigma). For corticosterone treatment, ten adult normal rats had ad libitum access to a drinking solution of 0.2 mg ml −1 corticosterone hemisuccinate on alternate days for 4 weeks. The average daily intake of corticosterone was ∼ 10–12 mg per rat. No difference in body weight or food intake was found between adult corticosterone-treated and CTL rats. For experiments on amblyopia recovery, MD was performed through eyelid suturing at postnatal day (P) 21. Once adult (P60) animals were divided in FR and CTL group, and after 2 weeks of dietetic regimen, RS was performed. The long-term deprived eye was re-opened using thin scissors, while the other eye was sutured. Great care was taken during the first week after RS to prevent inflammation or infection in the previously deprived eye through topical application of antibiotic and cortisone. In vivo electrophysiology At the end of the dietary regimen or drug treatment, the animals were anaesthetized with urethane (0.7 ml hg −1 ; 20% solution in saline; Sigma) by i.p. injection and placed in a stereotaxic frame. Body temperature was continuously monitored and maintained at ∼ 37 °C by a thermostated electric blanket during the experiment. An electrocardiogram was monitored. A hole was drilled in the skull, corresponding to the binocular portion of the primary visual cortex contralateral to the deprived eye. After exposure of the brain surface, the dura was removed, and a micropipette (2 MΩ) filled with NaCl (3 M) was inserted into the cortex 5 mm from intersection between sagittal- and lambdoid-sutures. We measured VA through both eyes using VEPs. To record VEPs, the electrode was advanced at a depth of 100 or 400 μm within the cortex. At these depths, VEPs had their maximal amplitude. Signals were band-pass-filtered (0.1–100 Hz), amplified and fed to a computer for analysis. Transient VEPs in response to abrupt contrast reversal (0.5 Hz) were evaluated in the time domain by measuring the peak-to-baseline amplitude and peak latency of the major negative component. Visual stimuli were horizontal sinusoidal gratings of different spatial frequencies presented on a monitor positioned 20 cm from the rat's eyes. VA was obtained by extrapolation to zero amplitude of the linear regression through the last four to five data points in a curve where VEP amplitude is plotted against log spatial frequency ( Supplementary Fig. S4 ). OD was assessed by calculating the ratio of VEP amplitudes recorded by stimulating the eye contralateral and ipsilateral to the visual cortex where recording was performed. Visual cortex LTP Brains from adult FR rats or CTLs were removed and immersed in ice-cold cutting solution containing (in mM): NaCl, 3.1 KCl, 1.0 K 2 HPO 4 , 4.0 NaHCO 3 , 2.0 MgCl 2 , 1.0 CaCl 2 , 10 HEPES, 1.0 ascorbic acid, 0.5 myo-inositol, 2.0 pyruvic acid and 1.0 kynurenate, pH 7.3. Slices (0.35 mm thick) of visual cortex were obtained using a vibratome. Slices were perfused at a rate of 2 ml min −1 with 32 °C oxygenated recording solution. The recording solution was composed as the cutting solution with the following differences (in mM): 130 NaCl, 5.0 dextrose, 1.0 MgCl 2 , 2.0 CaCl 2 , 0.01 glycine, no kynurenate. Electrical stimulation (100 μs duration) was delivered with a bipolar concentric stimulating electrode (FHC) placed at the border of the WM and layer VI. FPs in layer III were recorded by a micropipette (1–3 MΩ) filled with recording solution. Baseline responses were obtained every 30 s with a stimulation intensity that yielded a half-maximal response. After achievement of a 20 min stable baseline (FP amplitude within 15% of change and with no evident increasing or decreasing trends), θ-burst stimulation was delivered to induce LTP. Hippocampal LTP Brains from CTLs and FR adult rats were removed. Transverse hippocampal slices (400 μM) were cut and single slices were continuously perfused at 32 °C with the same solution used for visual cortex experiments. Field excitatory postsynaptic potential (fEPSPs) were recorded in stratum radiatum of CA1 hippocampal region. A concentric bipolar stainless steel electrode was placed in the stratum radiatum for stimulating the Schaeffer collateral afferents (0.1-ms pulse duration). Test stimuli were applied at a stimulus intensity that elicited an fEPSP amplitude that was ∼ 50% of maximum. LTP was induced by a high-frequency stimulation consisting of four 100-Hz trains applied with an interval of 5 min; stimulus width was 0.2 ms during the trains. In vivo brain microdialysis Adult rats were anaesthetized with avertin and stereotaxically implanted with stainless steel guide shafts above the binocular visual cortex, immediately after RS, at coordinates: 7.3 mm posterior to bregma, 4.4 mm lateral to the midsagittal suture and 1 mm ventral to the skull. After 4 weeks of differential rearing (under FR or not), in vivo sampling of dialysates was performed inserting a microdialysis probe into the guide shaft previously implanted. The probe was connected to a dialysis system pumping an artificial cerebrospinal fluid (CSF) (142 mM NaCl, 3.9 mM KCl, 1.2 mM CaCl 2 , 1 mM MgCl 2 , 1.35 mM Na 2 HPO 4 , pH 7.4) at a flow rate of 1 μl min −1 . After a stabilization period of 6 h, sampling was carried out. Six samples (20 μl each) were collected every 20 min along 2 h for each animal. Glutamate and GABA were measured by HPLC analysis [50] (see Supplementary Methods ). Western blot Brains were rapidly removed and frozen on dry ice. Visual cortices and hippocampi were dissected and proteins were extracted with lysis buffer (10 mM Tris, 1 mM EDTA, 2.5 mM sodium pyrophosphate, 1 mM β-glycerophosphate, 1 mM sodium orthovanadate, 1 mM phenylmethylsulfonylfluoride, 10 μg ml −1 aprotinin, 10 μg ml −1 leupeptin, 1% igepal CA-630). Supernatant was used for BDNF or GAD65 analysis and the pellet, containing the nuclear fraction, was further treated for histone analysis BDNF Protein extracts (25 μg) were separated by electrophoresis and blotted, and filters were incubated O/N at 4 °C with an antibody specific for BDNF (1:200; N-20, Santa Cruz) or with anti-β-tubulin (1:6,000; Sigma). Blots were then rinsed for 20 min in -Tween buffered saline (TTBS), incubated in HRP-conjugated anti-mouse or anti-rabbit (1:3,000 Bio-Rad), rinsed, incubated in enhanced chemiluminescent substrate (Bio-Rad) and exposed to film (Hyperfilm, Amersham Biosciences). The amount of BDNF protein was evaluated measuring the optical density (OD) of the BDNF band at 14 kDa and dividing it by the OD of β-tubulin band on the same filter at 50 kDa. GAD65 Visual cortex samples were taken from animals treated with corticosterone on alternate days or CTLs. Protein extracts (10 μg) were separated by electrophoresis and blotted, and filters were incubated O/N with an antibody anti-GAD 65/67 (1 μg ml −1 ; Chemicon) or with anti-β-actin (1:3,000; Abcam). The amount of GAD65 protein was evaluated measuring the OD of the GAD65 band at 65 kDa and dividing it by the OD of β-actin band on the same filter at 42 kDa. Histone acetylation Histone acetylation was evaluated by western blot as described in Putignano et al . [35] (see Supplementary Methods ). Immunohistochemistry Animals were perfused transcardially with phosphate-buffered saline (10 mM; PBS) followed by fixative (4% paraformaldehyde, 0.1 M sodium phosphate, pH 7.4). Brains were removed and post-fixed O/N in the same fixative at 4 °C, before being immersed in 30% sucrose. Coronal sections (40 μm) from the cortex were cut on a microtome and collected in PBS. BDNF and WFA Free-floating sections were incubated for 1 h in a blocking solution (10% BSA, 0.3% Triton X-100, in PBS), then O/N at 4 °C in a solution of chicken polyclonal anti-BDNF antibody (1:400, Promega) or a solution of biotin-conjugated lectin Wisteria Floribunda (10 μg ml −1 , Sigma). Primary antibodies were revealed with biotinylated donkey anti-chicken followed by ABC kit (Vector) and nickel-enhanced diaminobenzidine reaction for BDNF (1:200, Promega) or with an 1 h incubation in CY3-conjugated extravidin for WFA (1:500, Sigma). Sections were acquired at 20× imagnification (1,024×1,024 pixels) using a confocal microscope to analyse the number of positive cells. Positive cells were counted in fields of 700 μm width, centred in OcB1 and covering the entire thickness of the cortex. The counting analysis was performed blind to the rearing condition. For each animal, at least five Oc1B sections were analysed. GAD65 After the blocking step, sections were incubated O/N with monoclonal antibody anti-GAD65 (Chemicon, MAB351, 1:500, in 1% BSA, 0,2% Triton) and revealed with biotinylated secondary antibody goat anti-mouse IgG (1:200, Vector Laboratories) followed by incubation in cy3-conjugated extravidin (1:500, Sigma). Image acquisition and analysis was carried out according to the protocol described in Ciucci et al . [51] A total sample of 40–50 neurons were analysed for each cortex. All images acquisition and analysis were carried out in blind. Statistical analysis Statistical analysis was performed with SigmaStat. All values are expressed as the mean±s.e.m., and a two-tailed Student's t -test was used for pairwise comparison. One-way ANOVA, followed by a Holm–Sidak post hoc test, was used to compare more than two groups. Two-way ANOVA was used in the analysis of food intake and body weight or LTP experiments. Significance level was 0.05. How to cite this article: Spolidoro, M. et al . Food restriction enhances visual cortex plasticity in adulthood. Nat. Commun. 2:320 doi: 10.1038/ncomms1323 (2011).